A bacterial platform for fermentative production of plant alkaloids The secondary metabolites of higher plants include diverse chemicals, such as alkaloids, isoprenoids and phenolic compounds (phenylpropanoids and flavonoids). Although these compounds are widely used in human health and nutrition, at present they are mainly obtained by extraction from plants and extraction yields are low because most of these metabolites accumulate at low levels in plant cells. Recent advances in synthetic biology and metabolic engineering have enabled tailored production of plant secondary metabolites in microorganisms, but these methods often require the addition of expensive substrates. Here we develop an Escherichia coli fermentation system that yields plant alkaloids from simple carbon sources, using selected enzymes to construct a tailor-made biosynthetic pathway. In this system, engineered cells cultured in growth medium without additional substrates produce the plant benzylisoquinoline alkaloid, ( S )-reticuline (yield, 46.0 mg l −1 culture medium). The fermentation platform described here offers opportunities for low-cost production of many diverse alkaloids. The secondary metabolites of higher plants include diverse chemicals, such as alkaloids, isoprenoids and phenolic compounds (phenylpropanoids and flavonoids), which are produced from primary metabolites such as amino acids or acetyl-CoA ( Supplementary Fig. S1 ). Although these compounds are widely used in human health and nutrition, at present they are mainly obtained by extraction from plants. However, extraction yields are low because most of these metabolites accumulate at low levels in plant cells. There have been many attempts to use plant metabolic engineering to increase the amounts of secondary metabolites. However, it is very difficult to obtain the desired products because of the complex and strict regulation of their biosynthesis. Chemical synthesis has also been used to produce plant secondary metabolites; however, the complexity and chirality of these compounds have hampered the development of cost-effective methods. Recently, there has been increasing interest in microbial production of plant secondary metabolites by reconstructing their biosynthetic pathways in microorganisms [1] , [2] , [3] , [4] , [5] . Among these metabolites, isoprenoids are produced from acetyl-CoA in the mevalonate pathway or glyceraldehyde-3-phosphate and pyruvic acid in the 1-deoxy- D -xylulose-5-phosphate pathway ( Supplementary Fig. S1 ). The biosynthesis of isoprenoids is well characterized, and they have been produced by microbes in a simple growth medium [6] . The other major groups of secondary metabolites, that is, alkaloids and phenolic compounds, are derived from aromatic amino acids ( Supplementary Fig. S1 ). These compounds can be produced via microbial fermentation, but such systems require the addition of expensive precursor chemicals [7] , [8] , [9] , which makes these methods commercially unfeasible. Production of alkaloids and phenolic compounds from an inexpensive and readily available material has been one of the most important challenges for metabolic engineering of secondary metabolites [10] , [11] . Alkaloids are low-molecular-weight, nitrogen-containing compounds that are found in ~20% of plant species. They are very important in medicine because of their high biological activities. Most alkaloids are derived from amines produced by the decarboxylation of amino acids, such as histidine, lysine, ornithine, tryptophan and tyrosine. One of the largest and most diverse groups of pharmaceutically important alkaloids is the benzylisoquinoline alkaloids (BIAs). BIAs, which include the analgesic compounds morphine and codeine and the antibacterial agents berberine and palmatine, are produced through ( S )-reticuline from L -tyrosine. Thus, ( S )-reticuline is a main branch-point intermediate in the biosynthesis of many types of BIAs, and also acts as a non-narcotic building block that is useful in the development of novel antimalarial and anticancer drugs. In this study, we focused on the fermentative production of ( S )-reticuline in Escherichia coli grown in a simple medium without additional substrates. Here we constructed a bacterial platform for plant alkaloid production from simple carbon sources. In this platform, a tailor-made alkaloid biosynthetic pathway from L -tyrosine was constructed in L -tyrosine over-producing E. coli cells. The recombinant strain could produce 46.0 mg l −1 of ( S )-reticuline from glycerol, suggesting that the fermentation platform would enable low-cost production of many diverse alkaloids. Design of an artificial BIA biosynthetic pathway We have already succeeded in synthesizing reticuline from dopamine [7] . Thus, to obtain BIAs from a simple medium without the addition of dopamine, there are two additional steps that must be introduced: fermentative production of L -tyrosine and conversion of L -tyrosine to dopamine. We first generated an E. coli strain that over-produces L -tyrosine by amino-acid fermentation. This was accomplished by three steps of genetic engineering. An E. coli strain has disrupted the tyrR gene, the product of which represses the expression of genes involved in aromatic amino-acid biosynthesis [12] . In addition, the feedback-inhibition-resistant (fbr) 3-deoxy- D -arabino-heptulosonate-7-phosphate (DAHP) synthase (fbr-DAHPS: aroG fbr ) and fbr-chorismate mutase/prephenate dehydrogenase (fbr-CM/PDH: tyrA fbr ) are overexpressed in the shikimic acid pathway [13] . To increase metabolic flow into the shikimic acid pathway, phosphoenolpyruvate synthetase (PEPS: ppsA ) and transketolase (TKT: tktA ) [14] are exogenously introduced ( Fig. 1 ). Thus, the L -tyrosine over-producing E. coli strain contains a knockout mutation in tyrR and a plasmid expressing the aroG fbr , tyrA fbr , ppsA and tktA genes ( Supplementary Fig. S2 ). The engineered E. coli cells produced L -tyrosine in the medium at a yield of ~4.37±0.17 g l −1 (24.0±0.94 mM; average yield±standard deviation from three independent experiments), when glycerol was used as the carbon source. The overall yield of L -tyrosine, when glycerol was used as a carbon source, was 29.5% (molar ratio). By contrast, the wild-type E. coli cells produced low quantities of L -tyrosine in culture. 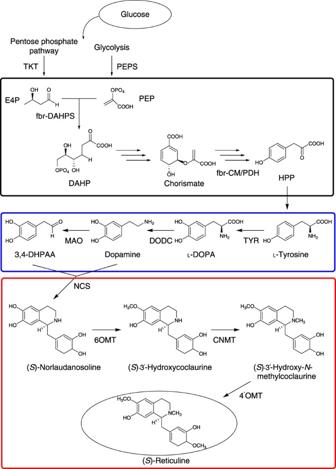Figure 1: Bacterial BIA biosynthetic pathway constructed inEscherichia colicells. ForL-tyrosine over-production, four enzymes (TKT, PEPS, fbr-DAHPS and fbr-CM/PDH) are overexpressed. Black box indicates the common aromatic pathway. The tailor-made biosynthetic pathway (blue) consisted of TYR, DODC and MAO. The plant biosynthetic pathway (red) was modified to circumvent the CYP80B reaction. CNMT, coclaurine-N-methyltransferase ofCoptis japonica(GenBank accession numberAB061863); DAHPS, 3-deoxy-D-arabino-heptulosonate-7-phosphate synthase (aroGfbr, GenBank accession numberJ01591); DODC, DOPA decarboxylase ofPseudomonas putida(GenBank accession numberAE015451); E4P, erythrose-4-phosphate; fbr, feedback-inhibition-resistant; fbr-CM/PDH, fbr-chorismate mutase/prephenate dehydrogenase (tyrAfbr, GenBank accession numberM10431); HPP, 4-hydroxyphenylpyruvate; MAO, monoamine oxidase ofMicrococcus luteus(GenBank accession numberAB010716); NCS, norcoclaurine synthetase ofC. japonica(GenBank accession numberAB267399); PEPS, phosphoenolpyruvate (PEP) synthetase (ppsA, GenBank accession numberX59381); TKT, transketolase (tktA, GenBank accession numberX68025); TYR, tyrosinase ofStreptomyces castaneoglobisporus(ScTYR containing tyrosinase and its adaptor protein, ORF378, GenBank accession numbersAY254101andAY254102) or tyrosinase ofRalstonia solanacearum(RsTYR,Rcs0337, GenBank accession numberAL646052); 3,4-DHPAA, 3,4-dihydroxyphenylacetaldehyde; 6OMT, norcoclaurine 6-O-methyltransferase ofC. japonica(GenBank accession numberD29811); 4′OMT, 3′-hydroxy-N-methylcoclaurine 4′-O-methyltransferase ofC. japonica(GenBank accession numberD29812). Figure 1: Bacterial BIA biosynthetic pathway constructed in Escherichia coli cells. For L -tyrosine over-production, four enzymes (TKT, PEPS, fbr-DAHPS and fbr-CM/PDH) are overexpressed. Black box indicates the common aromatic pathway. The tailor-made biosynthetic pathway (blue) consisted of TYR, DODC and MAO. The plant biosynthetic pathway (red) was modified to circumvent the CYP80B reaction. CNMT, coclaurine- N -methyltransferase of Coptis japonica (GenBank accession number AB061863 ); DAHPS, 3-deoxy- D -arabino-heptulosonate-7-phosphate synthase ( aroG fbr , GenBank accession number J01591 ); DODC, DOPA decarboxylase of Pseudomonas putida (GenBank accession number AE015451 ); E4P, erythrose-4-phosphate; fbr, feedback-inhibition-resistant; fbr-CM/PDH, fbr-chorismate mutase/prephenate dehydrogenase ( tyrA fbr , GenBank accession number M10431 ); HPP, 4-hydroxyphenylpyruvate; MAO, monoamine oxidase of Micrococcus luteus (GenBank accession number AB010716 ); NCS, norcoclaurine synthetase of C. japonica (GenBank accession number AB267399 ); PEPS, phosphoenolpyruvate (PEP) synthetase ( ppsA , GenBank accession number X59381 ); TKT, transketolase ( tktA , GenBank accession number X68025 ); TYR, tyrosinase of Streptomyces castaneoglobisporus (ScTYR containing tyrosinase and its adaptor protein, ORF378, GenBank accession numbers AY254101 and AY254102 ) or tyrosinase of Ralstonia solanacearum (RsTYR, Rcs0337 , GenBank accession number AL646052 ); 3,4-DHPAA, 3,4-dihydroxyphenylacetaldehyde; 6OMT, norcoclaurine 6- O -methyltransferase of C. japonica (GenBank accession number D29811 ); 4′OMT, 3′-hydroxy- N -methylcoclaurine 4′- O -methyltransferase of C. japonica (GenBank accession number D29812 ). Full size image The BIA synthetic pathway of plants has not been completely elucidated. 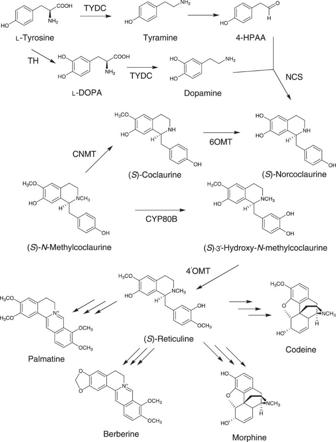Figure 2: Proposed plant biosynthetic pathway and genes involved in the biosynthesis of BIAs fromL-tyrosine to (S)-reticuline. CYP80B,N-methylcoclaurine 3′-hydroxylase; NCS, norcoclaurine synthase; TH, tyrosine hydroxylase; TYDC, tyrosine/dopa decarboxylase; 4-HPAA, 4-hydroxyphenylacetaldehyde; 6OMT, norcoclaurine 6-O-methyltransferase; 4′OMT, 3′-hydroxy-N-methylcoclaurine 4′-O-methyltransferase. The pathway to dopamine or 4-hydroxyphenylacetaldehyde (4-HPAA) from L -tyrosine is proposed in Figure 2 , but not all of the enzymes have been identified as yet. We originally designed an artificial pathway of reticuline synthesis using microbial enzymes. In plants and animals, L -DOPA is mainly synthesized from L -tyrosine by tyrosine hydroxylase (EC 1.14.16.2); however, tetrahydrobiopterin (BH4) is required as a cofactor for this reaction. E. coli cannot synthesize BH4; therefore, to convert L -tyrosine to L -DOPA, we chose tyrosinase (TYR; EC 1.14.18.1), which is unrelated to BIA biosynthesis. The TYRs from humans, Pholiota nameko and Streptomyces castaneoglobisporus were expressed in E. coli cells, and we examined their ability to convert L -tyrosine into L -DOPA. Only the TYR from S. castaneoglobisporus (ScTYR) successfully converted L -tyrosine into L -DOPA, and did not require unique cofactors other than copper and an adaptor protein (ORF378) [15] , [16] . When the selected TYR was expressed in the L -tyrosine over-producing E. coli strain, L -DOPA was produced in the medium at a yield of 293±5.9 mg l −1 . The conversion efficiency from L -tyrosine to L -DOPA was 6.19±0.13%. Figure 2: Proposed plant biosynthetic pathway and genes involved in the biosynthesis of BIAs from L -tyrosine to ( S )-reticuline. CYP80B, N -methylcoclaurine 3′-hydroxylase; NCS, norcoclaurine synthase; TH, tyrosine hydroxylase; TYDC, tyrosine/dopa decarboxylase; 4-HPAA, 4-hydroxyphenylacetaldehyde; 6OMT, norcoclaurine 6- O -methyltransferase; 4′OMT, 3′-hydroxy- N -methylcoclaurine 4′- O -methyltransferase. Full size image In our synthetic pathway, dopamine was synthesized from L -DOPA by the decarboxylation reaction ( Fig. 1 ). It is important that only L -DOPA undergoes decarboxylation. If other aromatic amines were produced by decarboxylation, monoamine oxidase (MAO; EC 1.4.3.4) would act on these amines to produce their corresponding aldehydes, which could then be accepted in the coupling reaction catalysed by norcoclaurine synthase (NCS; EC 4.2.1.78). Because MAO shows greater activity towards tyramine than dopamine, it was important to select an enzyme that specifically decarboxylates L -DOPA, not L -tyrosine; otherwise, MAO would act on tyramine produced by the decarboxylation of L -tyrosine, and the resulting 4-HPAA could then be accepted in the coupling reaction with dopamine catalysed by NCS. The coupling product, ( S )-norcoclaurine, is converted to ( S )- N -methylcoclaurine by norcoclaurine 6- O -methyltransferase (6OMT) and coclaurine- N -methyltransferase (CNMT). Because 3′-hydroxy- N -methylcoclaurine-4′- O -methyltransferase (4′OMT) has no ability to catalyse ( S )- N -methylcoclaurine [17] , the synthetic flow constructed in the cells terminated at ( S )- N -methylcoclaurine because of the lack of cytochrome P450 hydroxylase (CYP80B) in our system ( Figs 1 and 2 ). In the plant BIA biosynthetic pathway, tyrosine/DOPA decarboxylase (EC 4.1.1.25) catalyses the decarboxylation of L -tyrosine and L -DOPA to tyramine and dopamine, respectively [18] ( Fig. 2 ). For this reason, we selected the L -DOPA-specific decarboxylase (DODC; EC 4.1.1.28) from Pseudomonas putida strain KT2440, which exhibited a more than 10 3 -fold preference for L -DOPA than for other aromatic amino acids (Koyanagi T. et al ., in preparation). When the selected TYR and DODC were expressed in the L -tyrosine over-producing E. coli strain, dopamine was produced in the medium at a yield of ~260±22.7 mg l −1 . The conversion efficiency from L -tyrosine to dopamine was 7.08±0.62%, which was slightly improved compared with that from L -tyrosine to L -DOPA. The amount of melanin-like pigment in the culture medium of a dopamine-producing strain was lower than that in a L -DOPA-producing strain ( Supplementary Fig. S3 ). It was suggested that L -DOPA was converted into dopamine by DODC before the reaction of L -DOPA into dopaquinone. The Km value for L -DOPA of ScTYR was 8.1 mM (ref. 15 ). By contrast, the Km value for L -DOPA of P. putida DODC was 0.092 mM (Koyanagi T. et al ., in preparation). It was indicated that P. putida DODC dominates ScTYR in the reaction of L -DOPA, and the combination of TYR and DODC enables the conversion of L -tyrosine to dopamine with reducing dopaquinone formation. In the final step of the fermentative production of ( S )-reticuline, we combined the dopamine-producing pathway described above with the synthetic pathway from dopamine to ( S )-reticuline [7] . The genes encoding NCS and MAO were inserted into the pET-21d vector together with the genes for TYR and DODC. The genes for 6OMT, 4′OMT and CNMT were inserted into the pACYC184 vector ( Supplementary Fig. S2 ). The natural biosynthetic pathway in plants is not necessarily suitable for a microbial production system; therefore, our designed synthetic pathway differs from the original biosynthetic pathway. We carefully designed and optimized an artificial BIA pathway consisting of genes that were unrelated to the natural biosynthetic pathway ( Fig. 1 ). The newly designed pathway comprises one E. coli gene knockout, four overexpressed genes and eight exogenous genes. Our system uses selected enzymes to construct a single pathway from L -tyrosine to ( S )-norlaudanosoline. This system circumvents the complicated branched pathway and a potentially problematic CYP reaction in bacteria ( Figs 1 and 2 ). ( S )-Reticuline production from a simple carbon source Liquid chromatography–mass spectrometry (LC–MS) analysis showed that engineered E. coli cells produced up to 2.26 mg l −1 (average of 2.00±0.28 mg l −1 from three independent experiments) ( S )-reticuline from glucose in the culture medium ( Fig. 3a,b ). Without glucose, the yield of ( S )-reticuline was low (80 μg l −1 ), indicating that ( S )-reticuline was derived from a simple carbon source, glucose. The amount of ( S )-reticuline production was reduced to one-quarter in the wild-type E. coli cells with the synthetic pathway from L -tyrosine to ( S )-reticuline. This result confirmed that metabolic engineering of the aromatic amino-acid pathway effectively produced secondary metabolites from a simple carbon source. The growth rate of recombinant E. coli cells indicated that the intermediates in the reticuline biosynthetic pathway or ( S )-reticuline did not inhibit the growth of E. coli cells. In this system, ( S )-reticuline was produced by leaky expression of biosynthetic genes without induction by isopropyl-β- D -thiogalactoside (IPTG; Fig. 3c ), which substantially reduces production costs. When glycerol was used as the carbon source, ( S )-reticuline production increased up to 6.24 mg l −1 (average of 5.92±0.36 mg l −1 from three independent experiments) within 80 h ( Fig. 3d ), which was three times higher than the amount produced in the glucose-based medium. It was reported that glycerol is a more suitable carbon source than glucose for the production of shikimic acid and L -phenylalanine [19] , [20] . Therefore, it is likely that glycerol is also a more suitable carbon source for BIA production, as is the case for other products related to the shikimic acid pathway. The conversion efficiency from L -tyrosine to ( S )-reticuline was 0.150±0.01%, which is much lower than that for dopamine. To investigate the low conversion efficiency of ( S )-reticuline production, the amount of intermediate compounds, the expression levels of the biosynthetic genes ( TYR , ORF378 , DODC , MAO , NCS , 6OMT , CNMT and 4′OMT ), and the degradation of dopamine, norlaudanosoline and ( S )-reticuline in culture were examined. L -Tyrosine was not increased during growth, and other intermediate compounds ( L -DOPA, dopamine and intermediated BIAs) were not observed in the culture medium ( Supplementary Fig. S4 ), indicating that metabolic flow to reticuline was not interrupted. Reverse transcription PCR (RT–PCR) results indicated that all biosynthetic genes were expressed ( Fig. 4 ). The expression levels of plant genes ( NCS , 6OMT , CNMT and 4′OMT ) were low compared with microbial genes. The expression level of DODC was higher than that of TYR , which enables the conversion of L -DOPA to dopamine. The degradation analysis was carried out by adding substrates at a concentration close to that of the production yield to the culture medium. As a result, dopamine and norlaudanosoline were much more unstable than reticuline ( Supplementary Fig. S5 ). These observations, together with the fact that intermediated compounds were not accumulated ( Supplementary Fig. S4 ), indicated that the low yield of ( S )-reticuline from dopamine was attributed to the instability of dopamine and norlaudanosoline, and to a lesser extent, the inefficient conversion of L -tyrosine to L -DOPA. The increase in expression levels of plant genes could improve the usage efficiency of dopamine and norlaudanosoline. Although TYR catalyses the oxidation of L -tyrosine to L -DOPA, TYR also has the ability to convert L -DOPA or dopamine to its quinone derivative ( o -diphenolase), which is easily oxidized and polymerizes to form a melanin pigment. In our system, a melanin-like pigment was produced in the culture medium ( Supplementary Fig. S3 ). Therefore, we speculated that the instability of intermediate compounds might be attributed to o -diphenolase activity via TYR reactions. It has been reported that TYR from Ralstonia solanacearum (RsTYR) possesses low o -diphenolase activity [21] . This report prompted us to integrate RsTYR into our platform instead of ScTYR. As expected, the platform containing RsTYR produced up to 46 mg l −1 (average of 40.5±4.8 mg l −1 from three independent experiments) of reticuline, a yield approximately seven times higher than the platform using ScTYR ( Fig. 3d ). Because the dopamine-producing strain using RsTYR produced 1.05±0.05 g l −1 (6.85±0.30 mM) of dopamine, a yield almost four times higher than the dopamine-producing strain using ScTYR, the increased production ability of dopamine might contribute to increased reticuline production. 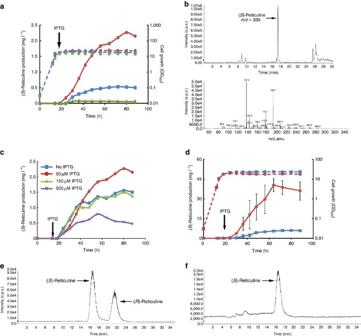Figure 3: Fermentative production of (S)-reticuline. (a) Time course of (S)-reticuline production inEscherichia colicultures.L-Tyrosine over-producingE. coli(red circles) or wild-type strains (blue squares) harbouringNCS-ScTYR-DODC-optMAO/pET-21d and6OMT-4′OMT-CNMT/pACYC184 were grown in a jar fermenter. In the case of anL-tyrosine over-producing strain, the culture was carried out in medium with (red circles) or without glucose (green triangles). Cell growth (broken lines with the same symbols as those for (S)-reticuline production) is represented as the optical density at 600 nm. The arrow indicates addition of IPTG (50 μM) at the indicated time. Data are representative of three independent experiments. (b) LC–MS/MS analysis of the reaction product from our system. Selected-ion monitoring (SIM) parameter:m/z=330 (reticuline). (c) Effect of IPTG concentration on fermentative production of (S)-reticuline in glucose-based medium. TheE. colistrain over-producingL-tyrosine and expressing reticuline biosynthetic genes was grown until the OD600was 10 before the addition of IPTG (arrow). No IPTG induction (blue squares), 50 μM (red circles), 150 μM (green triangles) or 500 μM IPTG (purple crosses). Data are representative of three independent experiments. (d) Fermentative production of (S)-reticuline in glycerol-based medium. A reticuline-producing strain using ScTYR (blue squares) or RsTYR (red circles) was cultured. The arrow indicates addition of IPTG (50 μM) at the indicated time. Cell growth (broken lines with the same symbols as those used for (S)-reticuline production) is represented as the optical density at 600 nm. The error bar indicates the standard deviation of three independent experiments. (e,f) Analysis of stereoselectivity of the reaction product towards (R,S)-reticuline. Authentic (R,S)-reticuline (e) and the reaction product in cultures ofE. colicells expressing biosynthetic genes (f) were analysed by LC–MS. SIM parameter:m/z=330 (reticuline). Figure 3: Fermentative production of ( S )-reticuline. ( a ) Time course of ( S )-reticuline production in Escherichia coli cultures. L -Tyrosine over-producing E. coli (red circles) or wild-type strains (blue squares) harbouring NCS-ScTYR-DODC -opt MAO /pET-21d and 6OMT-4′OMT-CNMT /pACYC184 were grown in a jar fermenter. In the case of an L -tyrosine over-producing strain, the culture was carried out in medium with (red circles) or without glucose (green triangles). Cell growth (broken lines with the same symbols as those for ( S )-reticuline production) is represented as the optical density at 600 nm. The arrow indicates addition of IPTG (50 μM) at the indicated time. Data are representative of three independent experiments. ( b ) LC–MS/MS analysis of the reaction product from our system. Selected-ion monitoring (SIM) parameter: m/z =330 (reticuline). ( c ) Effect of IPTG concentration on fermentative production of ( S )-reticuline in glucose-based medium. The E. coli strain over-producing L -tyrosine and expressing reticuline biosynthetic genes was grown until the OD 600 was 10 before the addition of IPTG (arrow). No IPTG induction (blue squares), 50 μM (red circles), 150 μM (green triangles) or 500 μM IPTG (purple crosses). Data are representative of three independent experiments. ( d ) Fermentative production of ( S )-reticuline in glycerol-based medium. A reticuline-producing strain using ScTYR (blue squares) or RsTYR (red circles) was cultured. The arrow indicates addition of IPTG (50 μM) at the indicated time. Cell growth (broken lines with the same symbols as those used for ( S )-reticuline production) is represented as the optical density at 600 nm. The error bar indicates the standard deviation of three independent experiments. ( e , f ) Analysis of stereoselectivity of the reaction product towards ( R , S )-reticuline. Authentic ( R , S )-reticuline ( e ) and the reaction product in cultures of E. coli cells expressing biosynthetic genes ( f ) were analysed by LC–MS. SIM parameter: m/z =330 (reticuline). 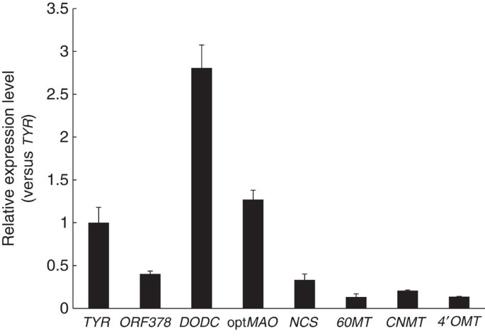Figure 4: Relative transcription level of the genes related to the reticuline production pathway. Total RNA was collected from a jar fermenter culture in glycerol-based Turbo Broth at 40 h post-inoculation. Transcription levels were determined by quantitative real-time PCR. The values represent the number of times the genes are expressed compared with expression of theTYRgene (set at 1.00). Results are presented as the average of six repetitions (triplicate reverse transcription reactions from two independent total RNA samples). Full size image Figure 4: Relative transcription level of the genes related to the reticuline production pathway. Total RNA was collected from a jar fermenter culture in glycerol-based Turbo Broth at 40 h post-inoculation. Transcription levels were determined by quantitative real-time PCR. The values represent the number of times the genes are expressed compared with expression of the TYR gene (set at 1.00). Results are presented as the average of six repetitions (triplicate reverse transcription reactions from two independent total RNA samples). Full size image Although NCS is an ( S )-form specific enzyme, reticuline was produced as a racemate in our previous system [7] because of a spontaneous condensation reaction involving dopamine and 3,4-dihydroxyphenylacetaldehyde to form ( R , S )-norlaudanosoline. The newly constructed system produced the ( S )-form exclusively ( Fig. 3e,f ). Furthermore, even when NCS was absent from our platform, which produced ( R , S )-norlaudanosoline by a spontaneous condensation reaction, ( R )-reticuline could not be detected ( Fig. 5a,b ). According to analysis of the reticuline production system from norlaudanosoline, ( R )-reticuline was detected only when a small amount of norlaudanosoline was added to the culture ( Fig. 5c–f ). These results led us to speculate that ( S )-reticuline accumulates because methyltransferases (6OMT, CNMT and 4′OMT) react to the ( S )-form in a superior manner to the ( R )-form, or that the ( R )-form ceases to be modified or degraded in E. coli cells. A larger amount of norlaudanosoline was available for reticuline production in our new platform compared with the dopamine-adding system [7] ; therefore, production of ( R )-reticuline was not observed in the newly constructed platform. The fermentative system developed in this study can produce optically active ( S )-reticuline rapidly (that is, in a few days) compared with fermentation systems using cultured plant cells or transgenic plants (months to years). 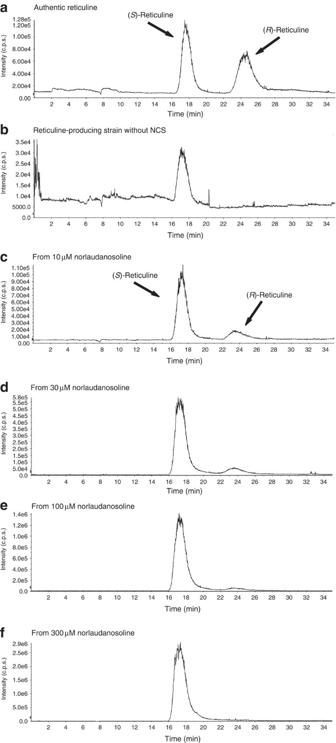Figure 5: Analysis of stereoselectivity of the reaction product towards (R,S)-reticuline. Authentic (R,S)-reticuline (a), the reaction product in the culture of the reticuline-producing strain without NCS (b), the reaction product in the culture of BL21DE3 cells harbouring6OMT-4′OMT-CNMT/pACYC184 (a plasmid for producing reticuline from norlaudanosoline) (c–f), were analysed by LC–MS. Selected-ion monitoring (SIM) parameter:m/z=330 (reticuline). BL21DE3 cells harbouring6OMT-4′OMT-CNMT/pACYC184 were grown in LB medium at 25 °C until the OD600reached 0.5. Then, 1 mM of IPTG and the indicated concentration, 10 μM (c), 30 μM (d), 100 μM (e) and 300 μM (f) of norlaudanosoline were added. Samples were collected at 12 h after induction. Figure 5: Analysis of stereoselectivity of the reaction product towards ( R , S )-reticuline. Authentic ( R , S )-reticuline ( a ), the reaction product in the culture of the reticuline-producing strain without NCS ( b ), the reaction product in the culture of BL21DE3 cells harbouring 6OMT-4 ′ OMT-CNMT /pACYC184 (a plasmid for producing reticuline from norlaudanosoline) ( c – f ), were analysed by LC–MS. Selected-ion monitoring (SIM) parameter: m / z =330 (reticuline). BL21DE3 cells harbouring 6OMT-4 ′ OMT-CNMT /pACYC184 were grown in LB medium at 25 °C until the OD 600 reached 0.5. Then, 1 mM of IPTG and the indicated concentration, 10 μM ( c ), 30 μM ( d ), 100 μM ( e ) and 300 μM ( f ) of norlaudanosoline were added. Samples were collected at 12 h after induction. Full size image The fermentation strategy for secondary metabolites described here requires cultivation of engineered cells in simple growth medium without additional substrates. Therefore, this system will drastically reduce the costs of producing scarce secondary metabolites. The glucose or glycerol used in this system is inexpensive and readily available, compared with the additional substrates that were required in previous microbial systems, such as dopamine or norlaudanosoline [7] , [8] . Although the overall yield of ( S )-reticuline in this system was low, we estimate that the production cost of ( S )-reticuline using this method would be much lower than that of previous microbial systems in terms of substrate costs. In addition to reduced production costs, another advantage of this system is the simple and effective purification procedure, which results in ( S )-reticuline with little contamination by other undesired BIAs. ( S )-Reticuline was purified from the culture medium using solid-phase extraction and high-performance liquid chromatography (HPLC; Supplementary Fig. S6 ). This procedure recovered more than 90% of purified ( S )-reticuline in two steps. A simple purification procedure resulting in high yields makes this production system economically viable. In plants, the secondary metabolite biosynthetic pathway is branched, complicated and difficult to reconstruct in a microbial production system. In this study, we first demonstrated the feasibility of fermentative production of a plant alkaloid from a simple carbon source, using selected enzymes to construct a tailor-made biosynthetic pathway in an L -tyrosine over-producing E. coli strain. We succeeded in ( S )-reticuline production by converting L -tyrosine to dopamine with a combination of selected TYR and DODC, and constructing a synthetic pathway from dopamine to a BIA skeleton using microbial MAO. ( S )-Reticuline is contained at low amount in natural plant, because it is an intermediated compound in BIA biosynthetic pathway. It was reported that ( S )-reticuline accumulated at high level in latex of transgenic opium poppy, which has antisense berberine bridge enzyme gene [22] . The amount of ( S )-reticuline accumulation was estimated ~320 mg per 1 l of latex over 60 days [22] , [23] . In the case of our platform, ( S )-reticuline accumulated about 40 mg per 1 l of culture medium within 3 days. In general, extraction of chemical compounds from plant sources has some problems, such as time cost, troublesome for collecting, difficult scale-up procedure. It was suggested that our bacterial platform would be more suitable for reticuline production than extraction procedure from plant sources. In our system, we produced ( S )-reticuline, which is a branch-point intermediate in the biosynthesis of many types of BIAs. Therefore, our bacterial platform can be used to produce ( S )-reticuline derivatives by chemosynthesis from ( S )-reticuline or by transforming the engineered strain with biosynthetic genes required for the target compound. Recently, two key enzymes in the morphine biosynthetic pathway, thebaine 6- O -demethylase and codeine O -demethylase, have been identified [24] . Therefore, the biosynthetic genes in the morphine biosynthetic pathway from ( R )-reticuline to morphine have been isolated and characterized completely. Morphine alkaloids are synthesized from ( S )-reticuline via ( R )-reticuline, which is a two-step isomerization reaction catalysed by 1,2-dehydroreticuline synthase and 1,2-dehydroreticulinium reductase [25] , [26] . Although the biosynthetic genes responsible for converting ( S )-reticuline to ( R )-reticuline have not been identified, our dopamine-adding system is able to produce reticuline as a racemate by using E. coli cells expressing reticuline biosynthetic genes without NCS [7] . In plant secondary metabolism, CYPs are one of the most important groups of biosynthetic enzymes. The expression and function of plant CYPs is potentially problematic in a microbial production system. However, the successful expression of plant CYPs in a microbial host such as E. coli , with modification of the amino-terminal region, has recently been reported [27] . Including these biosynthetic genes containing CYPs in our microbial fermentation system may achieve production of morphine alkaloids from simple carbon sources by ( R , S )-reticuline. Furthermore, because bacterial fermentation systems have advanced metabolic engineering for the production of amino acids, our platform could be further developed to produce other secondary metabolites. As an example, L -phenylalanine and L -tryptophan were easily over-produced in our system by overexpression of the branched pathway genes ( trp operon or pheA ) from chorismate to L -phenylalanine or L -tryptophan, respectively [28] . Indole alkaloids, which are the most structurally diverse alkaloids along with BIAs, are synthesized from L -tryptophan and secologanin, with several biosynthetic genes isolated and characterized [5] . The isolation of genes early in the pathway to secologanin enables our system to be expanded with respect to applications for metabolic engineering of many indole alkaloids ( Supplementary Fig. S1 ). Various phenolic compounds have been successfully produced from L -phenylalanine and L -tyrosine in microbial systems [9] . The fermentation system described here is easily applicable for metabolic engineering of phenolic compounds ( Supplementary Fig. S1 ). Many diverse secondary metabolites are derived from aromatic amino acids or acetyl-CoA; therefore, the fermentation platform described here illustrates a general strategy of metabolic engineering for the production of secondary metabolites, especially aromatic amino-acid derivatives. Combined with the fermentation platform for the production of isoprenoids [6] , our platform represents a significant advance in the metabolic engineering of secondary metabolites. Materials All synthetic genes were obtained from GenScript. ( R , S )-Norlaudanosoline was purchased from Acros Organics. L -Tyrosine, L -DOPA and dopamine were purchased from Sigma-Aldrich. ( R , S )-Reticuline was a gift from Mitsui Chemicals. Construction of expression vectors Construction of an E. coli strain over-producing L -tyrosine was achieved by the following steps: disruption of the tyrR gene [12] ; overexpression of fbr-DAHPS ( aroG fbr ) and fbr-CM/PDH ( tyrA fbr ) in the shikimic acid pathway [13] ; and increasing the metabolic flows into the shikimic acid pathway by overexpressing PEPS ( ppsA ) and TKT ( tktA ) [14] ( Fig. 1 ). We constructed an expression vector containing tyrA fbr , aroG fbr , tktA and ppsA . The genes tyrA fbr and aroG fbr cloned into pUC57 were purchased from GenScript and tyrA fbr was flanked by Nco I and Eco RI restriction enzyme recognition sites, and aroG fbr was fused to the T7 promoter. An Eco RI site was located upstream of the T7 promoter, and a Sac I site was located downstream of aroG fbr . The tktA and ppsA genes were amplified from genomic DNA of E. coli K-12 MG1655 using the primer sets NdeI-tktA-F and tktA-XhoI-R, and NdeI-ppsA-F and ppsA-XhoI-R, respectively ( Supplementary Table S1 ). After digestion with Nde I and Xho I, tktA and ppsA were individually cloned into pET-41a (Novagen) and pCOLADuet-1 (Merck), respectively. A DNA fragment containing the tyrA fbr gene was excised from tyrA fbr /pUC57 using Nco I and Eco RI, and then cloned into pCOLADuet-1. The Eco RI- Sac I fragment of aroG fbr /pUC57 was cloned into tyrA fbr /pCOLADuet-1, yielding the tyrA fbr - aroG fbr expression vector. We amplified tktA under the control of the T7 promoter from tktA /pET-41a using the primers 5Sac-T7 and 3NottktA ( Supplementary Table S1 ). These were then cloned into tyrA fbr - aroG fbr /pCOLADuet-1, generating tyrA fbr - aroG fbr - tktA /pCOLADuet-1. Finally, we digested ppsA /pCOLADuet-1 with Not I and Xho I to obtain a fragment containing the ppsA gene and the T7 promoter. This fragment was then cloned into tyrA fbr - aroG fbr - tktA /pCOLADuet-1, yielding tyrA fbr - aroG fbr - tktA - ppsA /pCOLADuet-1 ( Supplementary Fig. S2 ), and its sequence was confirmed. The norlaudanosoline synthetic pathway consists of four enzymes; TYR of S. castaneoglobisporus (ScTYR containing TYR and its adaptor protein, ORF378) or RsTYR ( Rcs0337 ), DODC of P. putida , MAO of Micrococcus luteus and NCS of Coptis japonica . In this study, we used a codon-optimized MAO (opt MAO ) and cloned it into a pGS-21a plasmid from GenScript. The MAO gene used previously ( NCS - MAO /pKK223-3) [7] was replaced by opt MAO driven by the T7 promoter. This was achieved by integrating the Bam HI- Hind III fragment of opt MAO and the T7 promoter generated by PCR using the primers 5Bam-T7 and 3oMAO ( Supplementary Table S1 ) into NCS - MAO /pKK223-3, generating NCS -opt MAO /pKK223-3. The PCR product for DODC ( Nde I- Bam HI fragment, obtained using the primers 5NdeDODC and 3BamDODC ( Supplementary Table S1 )) was ligated into the cognate site of pET-3a (Novagen). The DODC gene with the T7 promoter was amplified from DODC /pET-3a with the primers 5BamSacRVT7 and 3BamDODC ( Supplementary Table S1 ), and cloned into NCS-optMAO /pKK223-3. We purchased ScTYR or RsTYR cloned into pGS-21a from GenScript. The PCR product for ScTYR or RsTYR ( Sac I- Eco RV fragment, amplified using primers 5SacI-T7 and 3pGSEcoRV ( Supplementary Table S1 )) was ligated into the cognate site of NCS - DODC - optMAO /pKK223-3 yielding NCS-TYR-DODC-optMAO /pKK223-3. To compare production among lines harbouring different plasmid backbones, we generated a pET-21d (Novagen) plasmid-based vector. We amplified the fragment containing the T7 promoter fused to NCS from NCS-MAO /pKK223-3 (ref. 7 ) using the primers 5BglII-T7 and 3NCSBamSacRV ( Supplementary Table S1 ). The fragment was ligated into the Bgl II- Bam HI site of pET-21d. The Sac I- Hind III fragment for NCS - DODC -opt MAO /pKK223-3, containing DODC -opt MAO genes was ligated into NCS/pET-21d, generating NCS-DODC -opt MAO /pET-21d. Finally, the PCR product for TYR was ligated into the Sac I- Eco RV site of NCS - DODC -opt MAO /pET-21d, yielding NCS-TYR-DODC -opt MAO /pET-21d ( Supplementary Fig. S2 ). The line harbouring the pET-21d-based plasmid produced slightly higher levels of reticuline (0.14 versus 0.11 mg l −1 in the small-scale culture); therefore, we selected NCS-TYR-DODC -opt MAO /pET-21d as the expression plasmid for norlaudanosoline pathway enzymes. To construct the L -DOPA-producing strain, the Nde I- Xho I fragment of TYR /pGS-21a was cloned into the cognate site of pET-23a, yielding TYR /pET-23a. TYR and DODC ( Bam HI fragment of NCS-TYR-DODC -opt MAO /pET-21d) were cloned into pET-23a, yielding TYR - DODC /pET-23a. Construction of aromatic compound-producing strains The genetic design of the L -tyrosine over-producing strain is described by Lütke-Eversloh and Stephanopoulos [14] . The markerless deletion of tyrR , tyrR ∷ null strain, was constructed by PCR-based method [29] . BL21 (DE3) tyrR ∷ null was transformed with tyrA fbr - aroG fbr - tktA - ppsA /pCOLADuet-1, yielding the L -tyrosine over-producing strain. To construct the L -DOPA- and dopamine-producing strains, the L -tyrosine over-producing strain was transformed with TYR /pET-23a and TYR - DODC /pET-23a, respectively. To construct the reticuline-producing strain, the L -tyrosine over-producing strain was transformed with NCS - TYR - DODC -opt MAO /pET-21d and 6OMT-4′OMT-CNMT /pACYC184 (ref. 7 ; Supplementary Fig. S2 ). Fermentation conditions Cells were cultured overnight in liquid LB medium at 37 °C, then 10 ml of the cell culture was inoculated into 1 l of modified conventional medium (per litre: 47.6 g Turbo Broth (Athena Enzyme System), 1.6 g NH 4 Cl, 2.49 mg CuSO 4 ·5H 2 O, 3 g glucose or 5 g glycerol, and appropriate antibiotics (50 mg ampicillin, 25 mg kanamycin and 50 mg chloramphenicol). Cultures were grown at 25 °C in a 3-l jar fermenter (BMS-03PI, ABLE). The pH was maintained at 7.1 by automatic addition of 28% NH 4 OH and 1 M HCl. The agitation speed was 100 r.p.m. at the time of inoculation, and dissolved oxygen levels were allowed to fall to 10% of O 2 saturation with continuous air supply of 1 volume per volume per minute. The glucose concentration was maintained between 0.1 and 7 g l −1 by addition of 0.5 g ml −1 glucose solution. The glycerol concentration was maintained between 0.1 and 6 g l −1 by addition of 1 g ml −1 glycerol solution. If needed, an indicating concentration of IPTG was added to the culture when OD 600 reached 10 (glucose-based medium) or 15 (glycerol-based medium). Detection and quantification of chemical compounds Glucose in the culture medium was analysed by the mutarotase-glucose method using a Glucose CII Test Wako (Wako). Glycerol in the culture medium was analysed using a Glycerol Assay Kit (Cayman Chemical). To analyse aromatic compounds in the culture medium, except for reticuline and norlaudanosoline, cultures were collected and treated with 1 N HCl for solving crystallized tyrosine. After centrifugation, samples were analysed by HPLC equipped with a Discovery HS F5 column (Supelco). Compounds were separated on the column by increasing the concentration of acetonitrile from 3 to 20% in 10 mM ammonium formate (pH 3.0) at a flow rate of 0.5 ml min −1 . Elution of compounds was monitored by measuring absorbance at 280 nm. To measure reticuline and norlaudanosoline production, the culture medium was collected at various times, and proteins were precipitated with 2% trichloroacetate. The supernatant was analysed by LC–MS (3200 Q TRAP, Applied Biosystems Japan) after separation on an Agilent HPLC system (Agilent). The HPLC conditions were as follows: column, TSKgel ODS-80Ts (4.6×250 mm; Tosoh); solvent system, A: 0.1% acetic acid in water, B: 0.1% acetic acid in acetonitrile; gradient modes: 90% A (0–5 min), 90–60% A (5–20 min) and 10% A (20–30 min); flow rate, 0.5 ml min −1 at 40 °C. Reticuline was identified by comparison with authentic reticuline with regard to the fragmentation spectrum in LC–MS/MS. The amounts of reticuline and norlaudanosoline were estimated from standard curves using Analyst 1.4.1 software. Experiments were repeated three times. The stereoselectivity of reticuline was analysed by LC–MS after separation on an Agilent HPLC system. HPLC conditions were as follows: column, CHIRALCEL OD-H (4.6×250 mm, Daicel Chemical Industries); solvent system, hexane:2-propanol:diethylamine (72:28:0.1); flow rate, 0.55 ml min −1 at 40 °C. Quantitative RT–PCR analysis of synthetic pathway genes The reticuline-producing strain was grown on glycerol-based medium in a jar fermenter. IPTG (50 μM) was added to the culture when OD 600 reached 15. For total RNA extraction, cells were collected at 40 h post-inoculation. Total RNA was extracted using an RNeasy Mini kit (Qiagen). To eliminate contaminated DNA, we used DNaseI treatment system included in RNAqueous-4PCR Kit (Ambion). A total of 1.5 μg total RNA was used in reverse transcription reactions using a High Capacity cDNA Reverse Transcription Kit (Applied Biosystems). Relative RNA concentrations were determined by quantitative RT–PCR using a 7300 Real-time PCR system with TaqMan Gene Expression Assay (Applied Biosystems). Primers and probes were designed using Primer Express 1.5 software (Perkin-Elmer; Supplementary Table 1 ). The amount of mRNA was quantified against a standard curve using the C t value. Observation of aromatic compound degradation in culture The reticuline-producing strain was grown at 25 °C in Turbo Broth containing 10 μM of CuSO 4 and appropriate antibiotics without sugar. IPTG (50 μM) was added when OD 600 reached 10. At 12 h after IPTG induction, each substrate (final concentration: 0.5, 2 and 8 mM dopamine, 7.5, 30 and 120 μM norlaudanosoline or 7.5, 30 and 120 μM reticuline) was added to the culture. The additive reticuline was enzymatically synthesized from 0.45 mM of norlaudanosoline using a crude extract of BL21 (DE3) harbouring 6OMT-4′OMT-CNMT /pACYC184 (ref. 7 ). In all experiments, new synthesis of norlaudanosoline, mono- and di-methylated norlaudanosoline and reticuline were not observed. Purification of ( S )-reticuline ( S )-Reticuline was purified from culture medium with an Oasis HLB solid-phase extraction cartridge (Waters) and by HPLC. The cartridge was pre-equilibrated with water before loading the culture medium, washed with 5% methanol, and then ( S )-reticuline eluted with 100% methanol. The eluent was subjected to HPLC equipped with a TSKgel ODS-80Ts column. Peak fractions corresponding to ( S )-reticuline were collected, and the degree of refining confirmed by MS analysis. How to cite this article: Nakagawa, A. et al . A bacterial platform for fermentative production of plant alkaloids. Nat. Commun. 2:326 doi: 10.1038/ncomms1327 (2011).